IL-4 together with IL-1β induces antitumor Th9 cell differentiation in the absence of TGF-β signaling IL-9-producing CD4 + (Th9) cells are a subset of CD4 + T-helper cells that are endowed with powerful antitumor capacity. Both IL-4 and TGF-β have been reported to be indispensable for Th9 cell-priming and differentiation. Here we show, by contrast, that Th9 cell development can occur in the absence of TGF-β signaling. When TGF-β was replaced by IL-1β, the combination of IL-1β and IL-4 efficiently promoted IL-9-producing T cells (Th9 IL-4+IL-1β ). Th9 IL-4+ IL-1β cells are phenotypically distinct T cells compared to classic Th9 cells (Th9 IL-4+TGF-β ) and other Th cells, and are enriched for IL-1 and NF-κB gene signatures. Inhibition of NF-κB but not TGF-β-signaling negates IL-9 production by Th9 IL-4+IL-1β cells. Furthermore, when compared with classic Th9 IL-4+TGF-β cells, Th9 IL-4+IL-1β cells are less exhausted, exhibit cytotoxic T effector gene signature and tumor killing function, and exert a superior antitumor response in a mouse melanoma model. Our study thus describes an alternative pathway for Th9 cell differentiation and provides a potential avenue for antitumor therapies. Interleukin-9 (IL-9)-producing CD4 + T helper 9 (Th9) cells are a distinct subset of Th cells induced from naive CD4 + T cells by IL-4 together with transforming growth factor-β (TGF-β) cytokine signaling [1] , [2] . Although Th9 cell differentiation requires a regulatory network of transcription factors and Th9 cells express transcription regulators such as PU.1, IRF4, STAT6, GATA3, BATF, STAT5, HIF1α, and Foxo1 [3] , [4] , [5] , [6] , [7] , [8] , [9] , [10] , a unifying master transcription factor is still ambiguous. In addition to roles in allergic inflammation and autoimmune diseases, the most intriguing function of Th9 cells is their antitumor activity [4] , [10] , [11] , [12] . We were among the first to report antitumor features of Th9 cells [13] . Furthermore, increased physiological Th9 cell counts during nivolumab (anti-PD-1 antibodies (Abs)) treatment were associated with an improved clinical response among patients with metastatic melanoma [14] . More recently, we reported that Th9 cells represent a novel third paradigm for T cell therapy—they are less exhausted, fully cytolytic, and hyperproliferative, and only tumor-specific Th9 cells completely eradicated late-stage advanced tumors, a scenario more like that seen clinically [15] . Thus further work to elucidate the development of Th9 cells is warranted. Signals from IL-4 and TGF-β have been recognized as indispensable for Th9 cell differentiation, and neither IL-4 nor TGF-β is sufficient by itself to generate the Th9 cell transcriptional profile or to induce high amounts of IL-9 expression in T cells [6] , [10] , [16] . One study showed that Activin A, a member of TGF-β superfamily, may replicate the function of TGF-β in driving in vitro generation of Th9 cells [17] . However, the requirement for TGF-β signaling is unclear; one report has shown that IL-9 production from CD4 + T cells during a parasite infection is comparable between wild-type (WT) mice and TGF-βRII dominant-negative mice (which express a dominant-negative TGF-β receptor) [18] . Thus in the current study we sought to identify the potential of other cytokine combinations that may lead to Th9 cell priming and development. Here we report that Th9 cell differentiation can occur in the absence of TGF-β signaling. IL-4 in combination with IL-1β effectively induces generation of IL-9-producing CD4 + T cells (Th9 IL-4+IL-1β ), independent of endogenous TGF-β signaling. We demonstrate that the nuclear factor (NF)-κB pathway is required for IL-9 production in Th9 IL-4+IL-1β cells. Furthermore, Th9 IL-4+IL-1β cells promote antitumor immune responses in our experimental tumor-bearing model in vivo, achieving superior outcomes than those from classic Th9 IL-4+TGF-β cells. IL-4 together with IL-1β induces IL-9-producing CD4 + Th9 cells Classic Th9 cells are induced by IL-4 in combination with TGF-β cytokine signaling. Here we investigated whether TGF-β or IL-4 may be replaced by other cytokines to generate IL-9-producing CD4 + T cells. First, we primed naive tyrosinase-related protein (TRP)-1-specific CD4 + T cells with TRP-1 peptide-loaded antigen-presenting cells (APCs) by IL-4 in combination with other cytokines; we also generated other Th cell subsets Th1, Th2, Th17, and Th22 and classic Th9 IL-4+TGF-β cells as controls. IL-4 plus IL-1β, but not other cytokines, induced a significant amount of Il9 expression comparable to classic Th9 IL-4+TGF-β cells generated under conventional IL-4 and TGF-β conditions (Fig. 1a ). We also primed naive TRP-1-specific CD4 + T cells by TGF-β in combination with other cytokines. 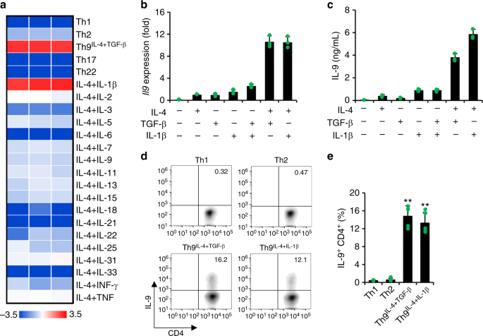Fig. 1 Interleukin (IL)-4 in combination with IL-1β promotes IL-9-producing CD4+T cell development. Naive CD4+CD62L+T cells were purified from the spleens of tyrosinase-related protein-1 mice and cocultured with irradiated antigen-presenting cells under polarized conditions as detailed in the Methods section (polarized in vitro for 3 days).aReverse transcriptase–PCR (RT-PCR) was performed to determine the expression ofIl9genes. Shown is the heatmap illustrating the relative expression ofIl9(data are log scaled) (n= 3).bRT-RCR analysis ofIl9expression in T cells primed with different cytokines as indicated (n= 3).cIL-9 production was measured by enzyme-linked immunosorbent assay in the supernatants of differentiated T cells in vitro (n= 3).d,eIntracellular staining showing the percentages of IL-9-producing cells in polarized T helper type 1 (Th1), Th2, classic Th9IL-4+ TGF-β, and Th9IL-4+IL-1βcells (n= 5). Representative data (d) and summarized results (e) are shown. Representative results of one from at least two repeated experiments are shown. Data are mean ± SD; **P< 0.01, compared with Th1 or Th2 cells, Student’sttest However, only TGF-β incorporated with IL-4 to promote Il9 gene expression, and no other cytokine appeared to replace the role of IL-4 (Supplementary Figure 1 ). These results suggest that the new cytokine milieu (IL-4+IL-1β) plays a crucial role and effectively induces IL-9-producing CD4 + cells. We further confirm that IL-4, IL-1β, or TGF-β is not sufficient to upregulate IL-9 expression at both the gene (reverse transcriptase–PCR (RT-PCR)) and protein (enzyme-linked immunosorbent assay (ELISA)) levels, whereas IL-4+IL-1β induces IL-9 expression comparable to the classic IL-4+TGF-β cocktail (Fig. 1b, c ). 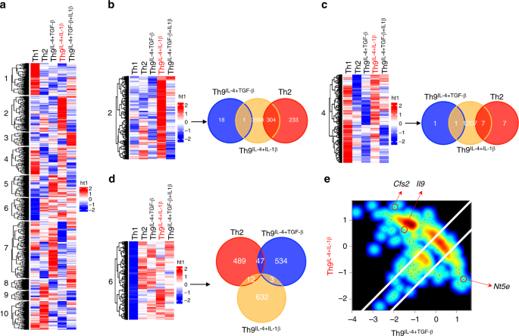Fig. 2 Th9IL-4+IL-1βcells have an identifiable transcriptional signature. Naive CD4+CD62L+T cells were purified from the spleens of tyrosinase-related protein-1 mice and cocultured with irradiated antigen-presenting cells under polarized conditions for 3 days, and RNA was extracted for gene array analysis.aHierarchical clustering of expression levels of 32,471 transcripts in T helper type 1 (Th1), Th2, classic Th9IL-4+TGF-β, Th9IL-4+IL-1β, and Th9IL-4+TGF-β+IL-1βcells. Cut-tree algorithm divided the transcripts into 10 clusters according to the distances between them defined by average method.bVenn diagrams displaying the number of upregulated genes of Th2, classic Th9IL-4+TGF-β, and Th9IL-4+IL-1βcells in cluster 2. The threshold for the upregulated genes is set asz-score = 0.9.cVenn diagrams showing the number of upregulated genes of Th2, classic Th9IL-4+TGF-β, and Th9IL-4+IL-1βcells in cluster 4. The threshold for the upregulated genes is set asz-score = 0.9.dVenn diagrams showing the number of upregulated genes of Th2, classic Th9IL-4+TGF-β, and Th9IL-4+IL-1βcells in cluster 6. The threshold for the upregulated genes is set asz-score = 0.9.eSpecific genes upregulated or downregulated by Th9IL-4+IL-1βcells versus classic Th9IL-4+TGF-β. Axis denotes the scaled expression levels represented byz-scores in the scatter plot.Csf2andIl9are uniquely upregulated (z-score is >1 and 0, respectively) in Th9IL-4+IL-1βcells, whereasNt5eis specifically upregulated in classic Th9IL-4+TGF-βcells withz-score >1 The concentration of IL-1β at 10 ng/ml was used thereafter because it is the optimal dose for IL-9 expression in Th9 IL-4+IL-1β cells (Supplementary Figure 2 ). 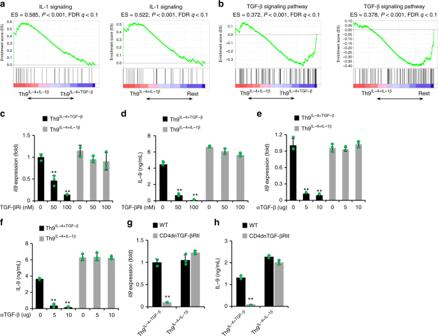Fig. 3 Differentiation of Th9IL-4+IL-1βcells is transforming growth factor (TGF)-β independent.a–fT cells differentiation and gene array data are the same as shown in Fig.2.aGene set enrichment analysis (GSEA) of Th9IL-4+IL-1βcells versus classic Th9IL-4+TGF-βcells or the Rest T helper (Th) cells for interleukin (IL)-1 signaling genes. Rest Th cells contain Th1, Th2, Th9IL-4+TGF-β, and Th9IL-4+TGF-β+IL-1βcells.bGSEA of Th9IL-4+IL-1βversus classic Th9IL-4+TGF-βcells or the Rest Th cells for TGF-β signaling genes.c,dReverse transcriptase–PCR (RT-PCR) analysis ofIl9transcriptional level (c) and enzyme-linked immunosorbent assay (ELISA) of IL-9 production in the supernatants (d) from TGF-βRi-treated classic Th9IL-4+TGF-βcells or Th9IL-4+IL-1βcells at the indicated concentrations (n= 3). TGF-βRi TGF-β receptor serine kinase inhibitor.e,fRT-PCR analysis ofIl9transcriptional level (e) and ELISA of IL-9 production in the supernatants (f) from αTGF-β-treated classic Th9IL-4+TGF-βcells or Th9IL-4+IL-1βcells at the indicated concentrations (n= 3). αTGF-β TGF-β monoclonal antibody (mAb).g,hNaive CD4+CD62L+T cells were purified from the spleens of wild-type (WT) mice or CD4dnTGF-βRII mice and cultured with plate-bound anti-CD3 mAbs and soluble anti-CD28 mAbs under polarized conditions, as detailed in the Methods section, for 3 days. RT-PCR analysis ofIl9transcriptional level (g) and ELISA of IL-9 production in the supernatants (h) of classic Th9IL-4+TGF-βcells and Th9IL-4+IL-1βcells from WT mice or CD4dnTGF-βRII mice after in vitro differentiation (n= 3). CD4dnTGF-βRII mice mice expressing a dominant-negative TGF-β receptor. Data are mean ± SD; **P< 0.01, Student’sttest. Representative results of one from two repeated experiments are shown In addition, Th9 IL-4+IL-1β and Th9 IL-4+TGF-β cells also produce a similar level of IL-10, which has been considered as another cytokine associated with Th9 cells (Supplementary Figure 3 ). The intracellular staining further supported the IL-9 production in Th9 IL-4+IL-1β cells (Fig. 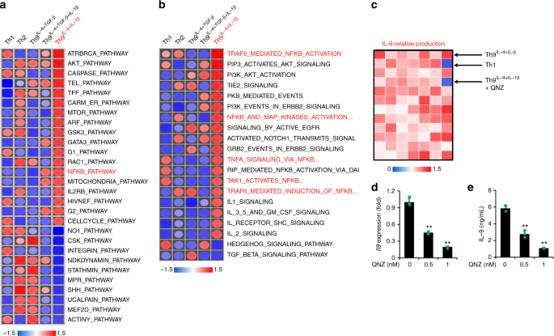Fig. 4 Nuclear factor (NF)-κB pathway is required for Th9IL-4+IL-1βcell differentiation. T cells differentiation and gene array data are the same as shown in Fig.2.a,bHeatmaps of enriched signaling of the most upregulated/downregulated pathways for T helper type 1 (Th1), Th2, classic Th9IL-4+TGF-β, Th9IL-4+IL-1β, and Th9IL-4+TGF-β+IL-1βcells.cInterleukin (IL)-9 production was measured by enzyme-linked immunosorbent assay (ELISA) in the supernatants of in vitro differentiated T cells. Shown is the heatmap of IL-9 relative production in the supernatants of Th1 and Th9IL-4+IL-1βcells and inhibitor-treated Th9IL-4+IL-1βcells (Kinase Inhibitor library, also see Supplementary Figure10a).d,eRT-PCR analysis ofIl9transcriptional level (d) and ELISA of IL-9 production in the supernatants (e) of QNZ-treated Th9IL-4+IL-1βcells at the indicated concentrations (n= 3). QNZ NF-κB pathway inhibitor. Data are mean ± SD; **P< 0.01, Student’sttest. Representative results from one of two repeated experiments are shown 1d, e ), whereas Th9 IL-4+IL-1β or Th9 IL-4+TGF-β cells produced limited IL-4, IL-5, or IL-13 (Supplementary Figure 4 ). Taken together, IL-4 with IL-1β is an alternative cytokine combination that efficiently induces IL-9-producing CD4 + cells. Fig. 1 Interleukin (IL)-4 in combination with IL-1β promotes IL-9-producing CD4 + T cell development. Naive CD4 + CD62L + T cells were purified from the spleens of tyrosinase-related protein-1 mice and cocultured with irradiated antigen-presenting cells under polarized conditions as detailed in the Methods section (polarized in vitro for 3 days). a Reverse transcriptase–PCR (RT-PCR) was performed to determine the expression of Il9 genes. Shown is the heatmap illustrating the relative expression of Il9 (data are log scaled) ( n = 3). b RT-RCR analysis of Il9 expression in T cells primed with different cytokines as indicated ( n = 3). c IL-9 production was measured by enzyme-linked immunosorbent assay in the supernatants of differentiated T cells in vitro ( n = 3). d , e Intracellular staining showing the percentages of IL-9-producing cells in polarized T helper type 1 (Th1), Th2, classic Th9 IL-4+ TGF-β , and Th9 IL-4+IL-1β cells ( n = 5). Representative data ( d ) and summarized results ( e ) are shown. Representative results of one from at least two repeated experiments are shown. Data are mean ± SD; ** P < 0.01, compared with Th1 or Th2 cells, Student’s t test Full size image The generation of Th9 IL-4+IL-1β cells is not limited to TRP-1-specific CD4 + T cells. 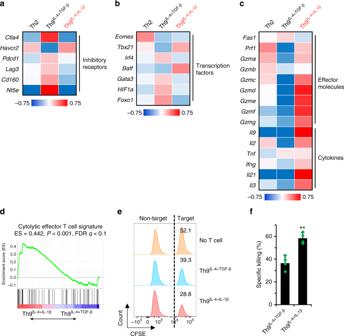Fig. 5 Th9IL-4+IL-1βcells exhibited antitumor activity in vitro. T cells differentiation and gene array data are the same as shown in Fig.2.aHeatmap illustrating the relative expression of exhaustion/inhibition markers as indicated (data are log scaled).bHeatmap illustrating the relative gene expression of transcription factors as indicated (data are log scaled).cHeatmap illustrating the relative gene expression (data are log scaled).dGene set enrichment analysis of classic Th9IL-4+TGF-βcells versus Th9IL-4+IL-1βcells for cytolytic effector T cell signature.e,fSpecific killing assay of tyrosinase-related protein-1 classic Th9IL-4+TGF-βor Th9IL-4+IL-1βwas performed against CFSEhigh-B16 tumor cells as target cells and CFSElow-MC38 tumor cells as a non-target control. An E:T ratio of 10:1 was used, and specific killing was determined after 48 h of coculture. Representative data (e) and summarized data (f) are shown (n= 4). Data are mean ± SD; **P< 0.01, Student’sttest. Representative results from one of two repeated experiments are shown We also used ovalbumin (OVA)-specific CD4 + T cells (from OT-II mice) and generated a similar IL-9-producing Th9 IL-4+IL-1β cells (Supplementary Figure 5 ). To determine in which cells, T cells and/or APCs, IL-1β signaling is required, we cocultured WT T cells and Il1r -deficient APCs or Il1r -deficient T cells and WT APCs. 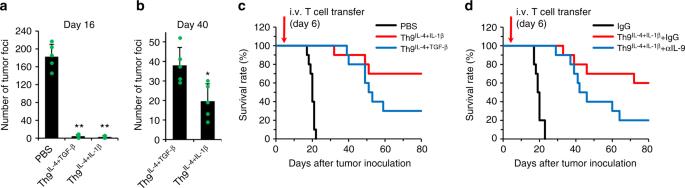Fig. 6 The antitumor activity of Th9IL-4+IL-1βcells in vivo. C57BL/6 mice were challenged with 1 × 105B16 cells delivered intravenously. T cells were differentiated as in Fig.2, and 1 × 106tyrosinase-related protein (TRP)-1 T cells were transferred on day 6 after tumor challenge.a,bTRP-1-specific classic Th9IL-4+TGF-βcells or Th9IL-4+IL-1βcells were transferred into tumor-bearing mice, tumor foci in the lung were counted on day 16 (a) or day 40 (b) after tumor inoculation (n= 5 mice/group).cThe survival rate of tumor-bearing mice with the indicated treatments (n= 10 mice).dThe survival rate of tumor-bearing mice with the indicated treatments (n= 10 mice). Control IgG or αIL-9 were injected intraperitoneally twice every week starting at 1 day before intravenous transfer of T cells. Data are mean ± SD; *P< 0.05, **P< 0.01, Student’sttest. Representative results from one of two repeated experiments are shown As shown in Supplementary Figure 6a, b , Il1r deficiency in T cells but not APCs abrogated IL-9 production of Th9 IL-4+IL-1β cells. In addition, IL-4+IL-1β is sufficient to induce IL-9 expression in naive CD4 + T cells stimulated with plate-bound αCD3/αCD28 mAbs (Supplementary Figure 6c, d ). Finally, in mice bearing lung metastatic B16-OVA tumors, Il1r deficiency or CD4 + T cell-depletion significantly impaired the IL-9 production of leukocytes isolated from the lung tumor tissues (Supplementary Figure 7 ), suggesting that IL-1β also contributes to the generation of IL-9-secreting T cells in vivo. Th9 IL-4+IL-1β cells display a distinct gene signature Next, we explored whether IL-4- and IL-1β-induced Th9 IL-4+ IL-1β cells represent a unique T cell subset compared with other known Th cells. We performed a microarray analysis comparing Th9 IL-4+IL-1β cells with Th1, Th2, classic Th9 IL-4+TGF-β cells, and Th9 IL-4+TGF-β+IL-1β cells (generated in the presence of TGF-β together with IL-4 and IL-1β, in which IL-1β serves a stimulator to further enhance the IL-9 expression from classic Th9 IL-4+TGF-β cells [19] , [20] ). Clustering analysis indicated that Th9 IL-4+ IL-1β cells have a gene signature that is distinct from any other four types of Th cells (Fig. 2a ). Gene clustering also identified three gene clusters (clusters 2, 4, and 6) enriched in these unique genes that are specifically upregulated in Th9 IL-4+IL-1β cells. These three clusters were further explored using commonality analysis [21] and overlap among the three cell types Th2, classic Th9 IL-4+TGF-β , and Th9 IL-4+IL-1β were analyzed by Venn diagrams. We detected 304, 7, and 12 overlapping transcriptional changes between Th9 IL-4+IL-1β cells and Th2 cells in clusters 2, 4, and 6, respectively; whereas only 1, 1, and 3 genes in clusters 2, 4, and 6, respectively, were identified as overlapping transcriptional changes between Th9 IL-4+IL-1β cells and classic Th9 IL-4+TGF-β cells (Fig. 2b–d ). Of note, these overlapping genes in clusters 2, 4, and 6 only account for ~about 6% of all unique genes in Th9 IL-4+ IL-1β cells, suggesting that they may represent a separate T cell phenotype. Next, we analyzed global gene expression in Th9 IL-4+IL-1β and classic Th9 IL-4+TGF-β cells. Th9 IL-4+ IL-1β cells possess >50% differentially expressed genes compared to classic Th9 IL-4+TGF-β cells (Fig. 2e ). Apart from increased Il9 expression, Th9 IL-4+IL-1β cells also express markedly increased Csf2 (the gene that encodes GM-CSF), which is reported to be a unique gene induced by IL-1β [22] , [23] . By contrast, classic Th9 IL-4+TGF-β cells show highly upregulated Nt5e , the gene specifically promoted by TGF-β [24] , [25] . Taken together, these data indicate that Th9 IL-4+IL-1β cells have an identifiable transcriptional signature that may result in unique functional properties. Fig. 2 Th9 IL-4+IL-1β cells have an identifiable transcriptional signature. Naive CD4 + CD62L + T cells were purified from the spleens of tyrosinase-related protein-1 mice and cocultured with irradiated antigen-presenting cells under polarized conditions for 3 days, and RNA was extracted for gene array analysis. a Hierarchical clustering of expression levels of 32,471 transcripts in T helper type 1 (Th1), Th2, classic Th9 IL-4+TGF-β , Th9 IL-4+IL-1β , and Th9 IL-4+TGF-β+IL-1β cells. Cut-tree algorithm divided the transcripts into 10 clusters according to the distances between them defined by average method. b Venn diagrams displaying the number of upregulated genes of Th2, classic Th9 IL-4+TGF-β , and Th9 IL-4+IL-1β cells in cluster 2. The threshold for the upregulated genes is set as z -score = 0.9. c Venn diagrams showing the number of upregulated genes of Th2, classic Th9 IL-4+TGF-β , and Th9 IL-4+IL-1β cells in cluster 4. The threshold for the upregulated genes is set as z -score = 0.9. d Venn diagrams showing the number of upregulated genes of Th2, classic Th9 IL-4+TGF-β , and Th9 IL-4+IL-1β cells in cluster 6. The threshold for the upregulated genes is set as z -score = 0.9. e Specific genes upregulated or downregulated by Th9 IL-4+IL-1β cells versus classic Th9 IL-4+TGF-β . Axis denotes the scaled expression levels represented by z -scores in the scatter plot. Csf2 and Il9 are uniquely upregulated ( z -score is >1 and 0, respectively) in Th9 IL-4+IL-1β cells, whereas Nt5e is specifically upregulated in classic Th9 IL-4+TGF-β cells with z -score >1 Full size image Th9 IL-4+IL-1β cell generation is independent of TGF-β signaling Endogenously produced TGF-β may contribute to IL-9 production from Th9 IL-4+IL-1β cells. To explore the contribution of endogenous TGF-β signaling, we first analyzed the IL-1β and TGF-β signaling pathway signatures in these Th cells. Using gene set enrichment analysis (GSEA), gene sets defined as in the IL-1-signaling pathway were imprinted in Th9 IL-4+IL-1β cells compared to classic Th9 IL-4+TGF-β cells and in all other Th cells (including Th1, Th2, and Th9 IL-4+TGF-β+IL-1β cells) (Fig. 3a ). As expected, TGF-β signaling signature was markedly downregulated in Th9 IL-4+IL-1β cells compared to classic Th9 IL-4+TGF-β cells or Rest Th cells (Fig. 3b ). Thus we hypothesize that TGF-β signaling is not required to produce IL-9 in Th9 IL-4+IL-1β cells. To test our hypothesis, we generated Th9 IL-4+IL-1β cells in the presence of TGF-β receptor serine kinase inhibitor (TGF-βRi). TGF-βRi treatment significantly downregulated Il9 gene expression and IL-9 secretion in the classic Th9 IL-4+TGF-β cells but did not change IL-9 production in Th9 IL-4+IL-1β cells (Fig. 3c, d ). To address the off-target potential of a chemical inhibitor, we also used anti-TGF-β antibody or CD4dnTGF-bRII mice. TGF-β neutralization abrogated IL-9 production in classic Th9 IL-4+TGF-β cells, while IL-9 production in Th9 IL-4+IL-1β cells was not affected (Fig. 3e, f ). Similar results were obtained when using naive TGF-βRII null CD4 + T cells isolated from CD4dnTGF-βRII mice. IL-9 production was markedly reduced in classic Th9 IL-4+TGF-β cells but not in Th9 IL-4+IL-1β cells generated from TGF-βRII null CD4 + T cells (Fig. 3g, h ). To exclude the possibility that IL-1β promotes the production of other TGF-β superfamily [17] and then indirectly induces IL-9 production, we checked the activation status of Smads in Th9 IL-4+IL-1β cells compared to classic Th9 IL-4+TGF-β cells. As shown in Supplementary Figure 8 , Th9 IL-4+TGF-β but not Th9 IL-4+ IL-1β cells had activated Smads, and as expected, Smad inhibitors had little impact on IL-9 production in Th9 IL-4+ IL-1β cells. Collectively, these results suggested that IL-4 plus IL-1β can effectively induce generation of Th9 cells without TGF-β signaling. Fig. 3 Differentiation of Th9 IL-4+IL-1β cells is transforming growth factor (TGF)-β independent. a – f T cells differentiation and gene array data are the same as shown in Fig. 2 . a Gene set enrichment analysis (GSEA) of Th9 IL-4+IL-1β cells versus classic Th9 IL-4+TGF-β cells or the Rest T helper (Th) cells for interleukin (IL)-1 signaling genes. Rest Th cells contain Th1, Th2, Th9 IL-4+TGF-β , and Th9 IL-4+TGF-β+IL-1β cells. b GSEA of Th9 IL-4+IL-1β versus classic Th9 IL-4+TGF-β cells or the Rest Th cells for TGF-β signaling genes. c , d Reverse transcriptase–PCR (RT-PCR) analysis of Il9 transcriptional level ( c ) and enzyme-linked immunosorbent assay (ELISA) of IL-9 production in the supernatants ( d ) from TGF-βRi-treated classic Th9 IL-4+TGF-β cells or Th9 IL-4+IL-1β cells at the indicated concentrations ( n = 3). TGF-βRi TGF-β receptor serine kinase inhibitor. e , f RT-PCR analysis of Il9 transcriptional level ( e ) and ELISA of IL-9 production in the supernatants ( f ) from αTGF-β-treated classic Th9 IL-4+TGF-β cells or Th9 IL-4+IL-1β cells at the indicated concentrations ( n = 3). αTGF-β TGF-β monoclonal antibody (mAb). g , h Naive CD4 + CD62L + T cells were purified from the spleens of wild-type (WT) mice or CD4dnTGF-βRII mice and cultured with plate-bound anti-CD3 mAbs and soluble anti-CD28 mAbs under polarized conditions, as detailed in the Methods section, for 3 days. RT-PCR analysis of Il9 transcriptional level ( g ) and ELISA of IL-9 production in the supernatants ( h ) of classic Th9 IL-4+TGF-β cells and Th9 IL-4+IL-1β cells from WT mice or CD4dnTGF-βRII mice after in vitro differentiation ( n = 3). CD4dnTGF-βRII mice mice expressing a dominant-negative TGF-β receptor. Data are mean ± SD; ** P < 0.01, Student’s t test. Representative results of one from two repeated experiments are shown Full size image NF-κB pathway is required for Th9 IL-4+IL-1β cell generation It is also important to determine what signaling pathway(s) is responsible for IL-9 production from Th9 IL-4+IL-1β cells. We first checked Irf1 , because it has been reported to regulate IL-9 production in Th9 IL-4+TGF-β+IL-1β cells [20] . However, we found no difference between IL-9 production in Th9 IL-4+IL-1β cells generated from naive CD4 + T cells isolated from WT mice or Irf1 -knockout mice (Supplementary Figure 9 ). To identify the potential pathway for IL-9 induction, we performed GSEA for enriched signaling(s) in Th9 IL-4+IL-1β cells (674 Reactome and 186 KEGG gene sets). As shown in Fig. 4a, b for the most upregulated/downregulated pathways, it seems that The NF-κB and AKT pathways were specifically activated in Th9 IL-4+IL-1β cells compared with other Th cells. Using a panel of chemicals containing 82 pathway inhibitors (Supplementary Figure 10a ), only the NF-κB pathway inhibitor QNZ significantly suppressed IL-9 production of Th9 IL-4+IL-1β cells (Fig. 4c ). We further confirmed that inhibition of IL-9 production of Th9 IL-4+IL-1β cells by QNZ was dose dependent (Fig. 4d, e ), whereas such effect on Th9 IL-4+TGF-β cells was moderate in comparison to that of Th9 IL-4+IL-1β cells (Supplementary Figure 10b-10d ). To further investigate the molecular requirement, we first used a luciferase reporter assay to examine which NF-κB family member(s) can bind and transcribe Il9 gene. We found RelA but not other members significantly enhanced the Il9 promoter transcriptional activity (Supplementary Figure 11a ). In addition, we detected a significantly increased binding of RelA to the Il9 promoter in Th9 IL-4+IL-1β cells by chromatin immunoprecipitation (ChIP) assay (Supplementary Figure 11b ). Finally, knockdown of RelA by small interfering RNA (siRNA) largely reduced IL-9 production in Th9 IL-4+IL-1β cells (Supplementary Figure 11c ). Therefore, these data suggest that activation of the NF-κB pathway is required for IL-9 production in Th9 IL-4+IL-1β cells. Fig. 4 Nuclear factor (NF)-κB pathway is required for Th9 IL-4+IL-1β cell differentiation. T cells differentiation and gene array data are the same as shown in Fig. 2 . a , b Heatmaps of enriched signaling of the most upregulated/downregulated pathways for T helper type 1 (Th1), Th2, classic Th9 IL-4+TGF-β , Th9 IL-4+IL-1β , and Th9 IL-4+TGF-β+IL-1β cells. c Interleukin (IL)-9 production was measured by enzyme-linked immunosorbent assay (ELISA) in the supernatants of in vitro differentiated T cells. Shown is the heatmap of IL-9 relative production in the supernatants of Th1 and Th9 IL-4+IL-1β cells and inhibitor-treated Th9 IL-4+IL-1β cells (Kinase Inhibitor library, also see Supplementary Figure 10a ). d , e RT-PCR analysis of Il9 transcriptional level ( d ) and ELISA of IL-9 production in the supernatants ( e ) of QNZ-treated Th9 IL-4+IL-1β cells at the indicated concentrations ( n = 3). QNZ NF-κB pathway inhibitor. Data are mean ± SD; ** P < 0.01, Student’s t test. Representative results from one of two repeated experiments are shown Full size image Th9 IL-4+IL-1β cells have a cytolytic effector signature Our group has a long-term interest in using tumor-specific Th9 cells as a novel therapeutic strategy for malignancies [7] , [13] , [15] , [26] , [27] . We next investigated whether these TGF-β signaling-independent Th9 IL-4+IL-1β cells are also potent antitumor T cells. Analysis of gene array data suggests that most exhaustion/inhibition markers are downregulated in Th9 IL-4+IL-1β cells compared to classic Th9 IL-4+TGF-β cells, including Ctla4 , Pdcd1 , Lag3 , and NT5e (Fig. 5a ). In particular, Th9 IL-4+IL-1β cells had greater expression of Eomes and Tbx21 (Fig. 5b ), transcriptional factors that suggest effector cell development [28] , [29] , [30] , and increased expression of a Grz panel ( Grza , Grzb , Grzc , Grzd , Grze , Grzf , Grzg ) and Prf1 (Fig. 5c ). Enhanced expression of cytokine genes, such as Il9 , Il2 , and Il21 , may also be involved in the superior antitumor functionality of Th9 IL-4+IL-1β cells. These observations prompted us to use GSEA to generate an enrichment plot for a cytolytic effector T cell gene signature. GSEA of the gene array data revealed that, as compared with the classic Th9 IL-4+TGF-β cells, the cytolytic effector T cell gene signature was significantly enriched in Th9 IL-4+IL-1β cells (Fig. 5d ), further suggesting that Th9 IL-4+IL-1β cells are also potent antitumor effector T cells. Indeed, tumor-specific Th9 IL-4+IL-1β cells displayed significantly higher tumor-specific killing activity compared to classic Th9 IL-4+TGF-β and Th2 cells in the in vitro cytolytic killing assay (Fig. 5e, f and Supplementary Figure 12a ). Fig. 5 Th9 IL-4+IL-1β cells exhibited antitumor activity in vitro. T cells differentiation and gene array data are the same as shown in Fig. 2 . a Heatmap illustrating the relative expression of exhaustion/inhibition markers as indicated (data are log scaled). b Heatmap illustrating the relative gene expression of transcription factors as indicated (data are log scaled). c Heatmap illustrating the relative gene expression (data are log scaled). d Gene set enrichment analysis of classic Th9 IL-4+TGF-β cells versus Th9 IL-4+IL-1β cells for cytolytic effector T cell signature. e , f Specific killing assay of tyrosinase-related protein-1 classic Th9 IL-4+TGF-β or Th9 IL-4+IL-1β was performed against CFSE high -B16 tumor cells as target cells and CFSE low -MC38 tumor cells as a non-target control. An E:T ratio of 10:1 was used, and specific killing was determined after 48 h of coculture. Representative data ( e ) and summarized data ( f ) are shown ( n = 4). Data are mean ± SD; ** P < 0.01, Student’s t test. Representative results from one of two repeated experiments are shown Full size image Th9 IL-4+IL-1β cells are potent antitumor T cells Next, we investigated whether tumor-specific Th9 IL-4+IL-1β cells possess antitumor capacity in vivo. We used the TRP-1 model of adoptive immunotherapy, which reproduces the clinical challenge of targeting gp75 tumor/self-antigen in the poorly immunogenic B16 melanoma model [15] . We transferred TRP-1-specific Th2 cells or classic Th9 IL-4+TGF-β cells or Th9 IL-4+IL-1β cells into B6 mice bearing 6-day established B16 lung metastatic murine melanoma. Analyzing the lung tumor foci on 16 days after tumor inoculation suggested that Th9 IL-4+IL-1β cells induced robust tumor clearance compared to phosphate-buffered saline (PBS) or Th2 cell-treated groups (Fig. 6a and Supplementary Figure 12b ), and Th9 IL-4+IL-1β cells also showed superior long-term (40 days) antitumor capacity compared to classic Th9 IL-4+TGF-β cells (Fig. 6b ). In addition, on day 80, 70% of Th9 IL-4+IL-1β cell-treated mice were alive versus 30% of mice receiving the classic Th9 IL-4+TGF-β cells (Fig. 6c ). Finally, IL-9 production from Th9 IL-4+IL-1β cells contributed to antitumor efficacy, since neutralization of IL-9 reduced survival of Th9 IL-4+IL-1β cell-treated mice (Fig. 6d ). Overall, our study indicates that Th9 IL-4+IL-1β cells are less exhausted T cells endowed with a cytotoxic T effector gene signature that can exert a superior antitumor response compared to classic Th9 IL-4+TGF-β cells. Fig. 6 The antitumor activity of Th9 IL-4+IL-1β cells in vivo. C57BL/6 mice were challenged with 1 × 10 5 B16 cells delivered intravenously. T cells were differentiated as in Fig. 2 , and 1 × 10 6 tyrosinase-related protein (TRP)-1 T cells were transferred on day 6 after tumor challenge. a , b TRP-1-specific classic Th9 IL-4+TGF-β cells or Th9 IL-4+IL-1β cells were transferred into tumor-bearing mice, tumor foci in the lung were counted on day 16 ( a ) or day 40 ( b ) after tumor inoculation ( n = 5 mice/group). c The survival rate of tumor-bearing mice with the indicated treatments ( n = 10 mice). d The survival rate of tumor-bearing mice with the indicated treatments ( n = 10 mice). Control IgG or αIL-9 were injected intraperitoneally twice every week starting at 1 day before intravenous transfer of T cells. Data are mean ± SD; * P < 0.05, ** P < 0.01, Student’s t test. Representative results from one of two repeated experiments are shown Full size image IL-4 and TFG-β have long been considered as the two essential cytokines to induce Th9 cell differentiation. Although additional cytokines (e.g., type I interferon (IFN), IL-1, IL-2, and IL-25) [9] , [19] , [20] , [31] , [32] and costimulatory signaling (e.g., OX40 and GITR) [33] , [34] , [35] enhance IL-9 production and Th9 cell differentiation, the studies were performed in the context of the standard cytokine milieu containing IL-4 and TGF-β. No study has thus far investigated whether IL-4 or TGF-β is replaceable for Th9 induction. In the current study, we, for the first time, found that Th9 cell development can occur in the absence of TGF-β signaling. When TGF-β has been replaced by IL-1β, differentiation of IL-9-producing T cells can be achieved. The presence of APCs may further facilitate Th9 IL-4+IL-1β cell differentiation, which may be a synergistic effect of APC-induced costimulation upon IL-1β stimulation. Our study provides new insight into Th9 cell development and may be crucial to understanding the signaling pathways that regulate Th9 cell fate and functions. Our new Th9 IL-4+IL-1β cells may represent a completely separate T cell phenotype compared to classic Th9 IL-4+TGF-β cells and other known Th subsets (Th1 and Th2 cells). This is supported by our gene array analysis of the global gene profile of Th9 IL-4+IL-1β cells. We distinguished 3 gene clusters with key gene features of Th9 IL-4+IL-1β cells, within which only ~6% of the unique genes are shared with Th2 or classic Th9 IL-4+TGF-β cells. When directly compared with the classic Th9 IL-4+TGF-β cells, the new Th9 IL-4+IL-1β cells display a large portion of differentially expressed genes. As expected, Th9 IL-4+IL-1β cells are imprinted with the IL-1 signaling pathway signature while the classic Th9 IL-4+TGF-β cells are enriched in the TGF-β signaling signature; this may be caused by the different priming cytokine signaling from IL-1β versus TGF-β. Our study also excluded the possibility that endogenously produced TGF-β or endogenous TGF-β superfamily member signaling in naive CD4 + T cells contribute to IL-9 production in Th9 IL-4+IL-1β cells. These studies indicate Th9 IL-4+IL-1β cells are phenotypically different from TGF-β-dependent classic Th9 IL-4+TGF-β cells. For development of classic Th9 IL-4+TGF-β cells, a large number of signaling molecules has been reported to be crucial for IL-9 transcription, including those downstream of IL-4 signaling (e.g., signal transducer and activator of transcription factor 6 (STAT6) and GATA3), TGF-β signaling (e.g., PU.1, TAK1, HIF1α, and SMAD), and common signaling/transcriptional factors in T cells (e.g., IRF4, BATF, STAT5, AKT, FOXO1, NFAT, and Notch) [7] , [8] , [10] , [36] . Thus it appears that IL-9 production or Th9 IL-4+TGF-β cell differentiation is not regulated by a master transcription factor but instead by a coordinated network. Using GSEA, we identified markedly enriched NF-κB and AKT pathway signatures in Th9 IL-4+IL-1β cells. After adding a panel of individual inhibitors at the beginning of the Th9 IL-4+IL-1β cell priming, we confirmed that IL-9 production depended on NF-κB. It has been reported that a variety of immunologically relevant ligands, like IL-1 family members, TNF family members, etc., can activate NF-κB pathway [37] . Our results suggest that NF-κB family member RelA is required for IL-9 production in Th9 IL-4+ IL-1β cells. However, RelB/p52 has been reported to be more active than RelA/p50 for IL-9 production in Th9 IL-4+TGF-β cells upon OX40 costimulation [33] . This may be a result of different epigenetic changes of Il9 gene promoter region in Th9 IL-4+IL-1β versus Th9 IL-4+TGF-β cells, which allows unique binding accessibilities for different NF-κB family members. Thus signaling through the NF-κB pathway, mainly RelA, is essential for Il9 transcription and IL-9 production in the Th9 IL-4+ IL-1β cells. Our long-term interest in Th9 cells is to explore their potential for cancer treatment [7] , [13] , [15] , [26] , [27] . Thus we investigated whether Th9 IL-4+IL-1β cells are also tumor killers. Interestingly, these cells display attractive antitumor effector T cell features, such as further downregulated expression of exhaustion markers and high enrichment in cytolytic effector T cell gene signatures, compared to classic Th9 IL-4+TGF-β cells. Direct comparisons of these two phenotypically distinct Th9 cells suggests that Th9 IL-4+IL-1β cells display higher tumor-specific cytotoxicity in vitro and improved tumor clearance in vivo compared to classic Th9 IL-4+TGF-β cells. Of note, Th9 IL-4+IL-1β cell-mediated therapeutic antitumor effects also require IL-9 production. Therefore, our study indicates that Th9 IL-4+IL-1β cells are less exhausted cytotoxic effector T cells and can exert an antitumor response superior to classic Th9 IL-4+TGF-β cells. In summary, we report for the first time that TGF-β is not indispensable for Th9 cell differentiation. IL-4 plus IL-1β effectively induced IL-9 production independently of TGF-β signaling. Our study further showed that the NF-κB pathway, mainly RelA, is required for IL-9 production of Th9 IL-4+IL-1β cells. Noticeably, tumor-specific Th9 IL-4+IL-1β cells are cytolytic effectors and endowed with robust antitumor function. Therefore, our findings confirm the current understanding underlying Th9 cell differentiation and provide an avenue for a potentially more powerful weapon for cancer immunotherapy. Mice C57BL/6, B6.Cg-Tg(Cd4-TGFBR2)16Flv/J, B6.129S2- Irf1 tm1Mak /J, B6.Cg-Tg(TcraTcrb)425Cbn/J, B6.129S7- Il1r1 tm1Imx /J, and B6.Cg- Rag1 tm1Mom Tyrp1 B-w Tg(Tcra,Tcrb)9Rest/J mice were purchased from The Jackson Laboratory. Male and female 6–8-week-old mice were used for each animal experiment. All experiments complied with protocols approved by the Institutional Animal Care and Use Committee at the Wake Forest School of Medicine. Cell lines B16 melanoma cell line was purchased from ATCC; MC-38 cell line was a gift from Dr.Patrick Hwu, MD Anderson Cancer Center. Cells were cultured in Iscove’s Modified Dulbecco’s Medium (Invitrogen) or RPMI 1640 Medium (Invitrogen) supplemented with 10% heat-inactivated fetal bovine serum (ThermoFisher Scientific), 100 U/ml penicillin-streptomycin, and 2 mM L-glutamine (both from Invitrogen). Reagents TGF-β receptor serine kinase inhibitor TGF-βRi (Cat#616452) was purchased from Millipore. NF-κB inhibitor QNZ (Cat#sc-200675) was purchased from Santa Cruz Biotechnology. Smad3 inhibitor SIS3 (Cat#S7959) and Smad2 inhibitor LY2109761 (Cat#S2704) were purchased from Selleckchem. The major histocompatibility complex (MHC) class II-restricted TRP-1 106–130 peptides (SGHNCGTCRPGWRGAACNQKILTVR) and the MHC class II-restricted OT II 323–339 peptides (ISQAVHAAHAEINEAGR) were purchased from GenScript. Mouse IL-4-neutralizing antibody (clone 11B11), mouse IFN-γ-neutralizing antibody (clone XMG1.2), mouse IL-9-neutralizing antibody (clone 9C1), mouse CD4 depletion antibody (clone GK1.5), and TGF-β-neutralizing antibody (clone 1D11.16.8) were purchased from BioXcell. Mouse cytokine IL-1β, IL-4, IL-6, IL-12, and TNF and human IL-2 and TGF-β were purchased from R&D Systems. Chemical inhibitor Panel (Enzo, SCREEN-WELL® Kinase Inhibitor library, Cat#BML-2832-0100; also see Supplementary Figure 7a ). In vitro Th cell differentiation Naive CD4 + CD62L + T cells were purified from the spleens of TRP-1 or OT II mice by isolation kit (STEMCELL Technologies, Cat#19765) according to the manufacturer’s protocol. TRP-1-specific naive CD4 T cells were cultured for 3 days with irradiated T cell-depleted splenic APCs from C57BL/6 mice in the presence of TRP-1 106-130 peptide (5 μg/ml) or OT II 323–339 peptides (5 μg/ml). Th1 polarized medium was supplemented with IL-2 (100 U/ml), IL-12 (5 ng/ml), and anti-IL-4 mAbs (10 μg/ml). Th2 polarized medium was supplemented with IL-2 (100 U/ml), IL-4 (10 ng/ml) and anti-IFN-γ mAbs (10 μg/ml). Th17 polarized medium was supplemented with IL-6 (30 ng/ml), TGF-β (2.5 ng/ml), and anti-IFN-γ mAbs (10 μg/ml). Th22 polarized medium was supplemented with IL-6 (10 ng/ml), TNF (5 ng/ml), and anti-IFN-γ mAbs (10 μg/ml). Th9 TGF-β+IL-4 polarized medium was supplemented with IL-4 (10 ng/ml), TGF-β (1 ng/ml), and anti-IFN-γ mAbs (10 μg/ml). Th9 IL-4+TGF-β+IL-1β polarized medium was supplemented with IL-4 (10 ng/ml), TGF-β (1 ng/ml), IL-1β (10 ng/ml), and anti-IFN-γ mAbs (10 μg/ml). Th9 IL-4+IL-1β polarized medium was supplemented with IL-4 (10 ng/ml), IL-1β (10 ng/ml, or used at the indicated concentrations), and anti-IFN-γ mAbs (10 μg/ml). In some experiments, naive CD4 + CD62L + T cells were activated as indicated in the polarized condition with plate-bound anti-CD3 mAbs (1.5 μg/ml, clone 17A2, eBioscience) and anti-CD28 mAbs (0.75 μg/ml, clone 37.51, eBioscience). In some experiments, antibody or inhibitor was added at the beginning of the T cell cultures. Real-time PCR Total RNA was extracted from cultured T cells using the RNeasy Mini Kit (Qiagen), followed by cDNA synthesis with the High-Capacity cDNA Reverse Transcription Kit (Applied Biosystems). RT-PCR was conducted with SYBR Select Master Mix (Applied Biosystems). Expression was normalized to the expression of the housekeeping gene Gapdh . Il9 forward: 5’-ATGTTGGTGACATACATCCTTGC-3’, Il9 reverse: 5’-TGACGGTGGATCATCCTTCAG-3’; Irf1 forward: 5’-AGGCATCCTTGTTGATGTCC-3’, Irf1 reverse: 5’-AATTCCAACCAAATCCCAGG-3’; and Gapdh forward: 5’-TTGATGGCAACAATCTCCAC-3’, Gapdh reverse: 5’-CGTCCCGTAGACAAAATGGT-3’. Flow cytometry After culture for 3 days, differentiated Th cells were restimulated for 5 h with TRP-1 peptide-loaded APC or phorbol myristate acetate (50 ng/ml; Sigma-Aldrich) and ionomycin (500 ng/ml; Sigma-Aldrich) in the presence of a protein transport inhibitor (GolgiPlug, BD Biosciences). Then cell surface markers were stained in flow cytometry staining buffer for 30 min on ice after Fc blocking, followed by staining for intracellular cytokines with the BD Fixation/Permeabilization Solution Kit. The results were analyzed using a fluorescence-activated cell sorter (FACS) Fortessa flow cytometer. αCD4 (clone RM4-4, 1:100), αIL-9 (clone RM9A4, 1:100), αIL-4 (clone 11B11, 1:100), and αIL-10 (clone JES5-16E3, 1:100) were from BioLegend; αIL-13 (clone eBio13A, 1:100) from ThermoFisher; αp-Smad-3 (clone O72-670, 1:50) from BD; and αp-Smad-5 (clone 41D10, 1:800) from CST. Enzyme-linked immunosorbent assay After 72 h of polarization, cell culture supernatants were tested by ELISA for mouse IL-9 (ThermoFisher) or IL-10 (ThermoFisher) or IL-5 (ThermoFisher) according to the manufacturer’s protocol. RNA interference of RelA siRNA targeting RelA and non-specific siRNA were purchased from ThermoFisher and transfected into T cells by Lipofectamine RNAiMAX Transfection Reagent (ThermoFisher) [38] . Luciferase reporter assay Mouse Il9 promoter (from −895 to +5) was subcloned into pGL4.10 basic vector (Promega). 293T cells were transiently transfected 24 h with reporter plasmids along with expression vectors [15] for RelA, RelB, c-Rel, p50, and p52 or control vector by Lipofectamine 2000 (Invitrogen). Luciferase was measured with the Dual-Luciferase Reporter Assay System according to the manufacturer’s instructions (Promega). ChIP assay SimpleChIP Plus Enzymatic Chromatin IP kits (Cell Signaling Technology) were used for ChIP assays according to the manufacturer’s protocol. For the ChIPn, anti-RelA and isotype-matched control antibody were purchased from Cell Signaling and used at a 1:50 dilution. The DNAs were analyzed by RT-PCR with the following primer set surrounding the RelA-binding site at the Il9 promoter region. ChIP primers: Forward: 5’-GCACTGGGTATCAGTTTGATG-3’, Reverse: 5’-CTCAGTCTACCAGCATCTTCC-3’. Values were subtracted from the amount of IgG control and were normalized to the corresponding input control. Fractionation of the lung C57BL/6 WT mice or Il1r KO mice were challenged with 1 × 10 5 B16-OVA melanoma cells. Mice were intraperitoneally (i.p.) given control IgG or αCD4-depletion mAbs (clone GK1.5, 200 μg/mice) on days 8 and 11 and then sacrificed on day 14. Lung tumor tissues were digested with 1 mg/ml of collagenase D (Roche) for 30 min at 37 °C and then with 0.01 mM EDTA (Sigma-Aldrich) for 5 min, to prevent aggregates. The cells were collected using Ficoll (GE Healthcare) density gradient centrifugation and the middle section of the gradient was enriched for leukocytes. In vitro cytotoxicity assay B16 target cells for TRP-1 CD4 + T cells were labeled with 5 µM carboxyfluorescein succinimidyl ester (CFSE), whereas MC38 nontarget cells were labeled with 0.25 µM CFSE as the control. B16 target (CFSE high ) or MC38 nontarget (CFSE low ) cells were incubated with PBS control, TRP-1-specific Th2 cells, TRP-1-specific classic Th9 IL-4+TGF-β cells, or TRP-1-specific Th9 IL-4+IL-1β cells. An E:T ratio of 10:1 was used, and specific killing was determined after 48 h of coculture. After coculture, CFSE + cells from each target and control well were mixed and analyzed by FACS. The percentage of specific lysis was calculated as follows: (1 − R × M2/M1) × 100, where M1 = non-target events, M2 = target events, and R = M1 in untreated group/M2 in untreated group. Tumor model and adoptive transfer To establish the 6-day established murine lung metastatic B16 melanoma model, mice were injected intravenously (i.v.) with 1 × 10 5 B16 tumor cells. For adoptive transfer experiments, mice were injected i.v. with 1 × 10 6 TRP-1-specific Th2, Th9 IL-4+TGF-β , or Th9 IL-4+IL-1β cells 6 days after tumor cell inoculation. Control IgG or α-IL-9 were injected i.p. twice every week starting at 1 day before i.v. transfer of T cells. At days 16 or 40 after tumor inoculation, mice were sacrificed for measurement of metastatic lung foci. All lung lobes were evaluated under a tissue-dissecting microscope. Mice were euthanized by using CO 2 asphyxiation and followed by cervical dislocation if any of the following symptoms appear: (1) weight loss of ≥20% of baseline body weight; (2) mice display significant lameness and disability in moving. Microarray analysis Total RNA was extracted with the RNeasy Mini Kit (Qiagen) from 3-day cultured Th1, Th2, classic Th9 IL-4+TGF-β , Th9 IL-4+IL-1β , and Th9 IL-4+TGF-β+IL-1β cells. RNA samples were sent to the Case Western Reserve University Genomic Core for quality evaluation using an Agilent Bioanalyzer. Samples with intact 18S and 28S ribosomal RNA bands with RNA integrity number >8.5 were processed for microarray analysis performed with a Mouse Gene 2.0 ST Kit at the Case Western Reserve University Genomic Core. GSEA was implemented using newly generated gene expression profiles of the five cell types and downloaded GSEA software (gsea-v3.0, http://software.broadinstitute.org/gsea/downloads.jsp ). P values were calculated with Kolmogorov–Smirnov test (threshold = 0.01). The false discovery rate, q value, is the estimated probability that a gene set with a given NES represents a false positive finding. The threshold for q value in GSEA is 0.25. Gene sets for the mature effector were derived from a publicly available study of the genes differentially expressed by more than two-fold in quaternary versus primary cells [39] . Venn diagram analysis based on Cut-tree algorithm To compare our Th9 IL-4+IL-1β cells with other cells, including known Th9 (Th9 IL-4+TGF-β ), and another Th9 cell induced by three molecules (Th9 IL-4+TGF-β+IL-1β ), and Th1 and Th2 cells, we utilized un-supervised hierarchical clustering [39] to cluster all genes in the microarray data into 10 clusters. Clusters 1–10 were identified by Cut-tree algorithm using the same distance method of average as hierarchical clustering [39] . Clusters 2, 4, and 6 showing Th9 IL-4+IL-1β -specific genes (for gene lists, see Supplementary data 1 , 2 , 3 ) were taken for commonality analysis by Venn graph [21] . The overlaps among the three cell types Th2, classic Th9 IL-4+TGF-β , and Th9 IL-4+IL-1β were analyzed by Venn diagram. The threshold for the upregulated genes for clusters 2, 4, and 6 is z -score = 0.9, where z -score is the scaled value of each gene across the 5 cell types. Hierarchical clustering was analyzed by complexheatmap using R and Venn diagram analysis was implemented by VennDiagram in R ( https://www.r-project.org/ ). Statistical analyses For statistical analysis, Student’s t test was used. A P value <0.05 was considered statistically significant. Results are presented as mean ± standard deviations (SD). Reporting Summary Further information on experimental design is available in the Nature Research Reporting Summary linked to this article.